A magnetic compass aids monarch butterfly migration Convincing evidence that migrant monarch butterflies ( Danaus plexippus ) use a magnetic compass to aid their fall migration has been lacking from the spectacular navigational capabilities of this species. Here we use flight simulator studies to show that migrants indeed possess an inclination magnetic compass to help direct their flight equatorward in the fall. The use of this inclination compass is light-dependent utilizing ultraviolet-A/blue light between 380 and 420 nm. Notably, the significance of light <420 nm for inclination compass function was not considered in previous monarch studies. The antennae are important for the inclination compass because they appear to contain light-sensitive magnetosensors. For migratory monarchs, the inclination compass may serve as an important orientation mechanism when directional daylight cues are unavailable and may also augment time-compensated sun compass orientation for appropriate directionality throughout the migration. During the fall, eastern North American monarch butterflies ( Danaus plexippus ) migrate south from their northern range to overwinter in sites atop the mountains of Michoacán in central Mexico [1] , [2] , [3] . Monarchs use an antenna-based time-compensated sun compass to navigate during this long journey [4] , [5] , [6] , in which eye-sensed directional daylight cues (for example, sun azimuthal position) are integrated in the sun compass found in the midbrain central complex area [7] , [8] and time compensated by antennal circadian clocks [9] , [10] . Curiously, during the absence of directional daylight cues that precludes the use of the time-compensated sun compass (for example, overcast sky conditions), migrants have been observed flying in the expected southern migratory direction during the fall migration [11] , suggesting that migrants might also use a magnetic compass to help guide directionality. We now show that migratory monarch butterflies have an inclination magnetic compass that allows them to orient in the proper southern direction during the fall migration. The inclination compass is light dependent, using light in the ultraviolet-A/blue spectral range. Relevant light-sensitive magnetosensors appear to reside in the antennae, and the inclination compass functions at Earth-strength magnetic fields. The inclination compass is an essential orientation mechanism that migrants can use when directional skylight cues are unavailable, and it may also augment time-compensated sun compass orientation. Migrant monarchs can use a magnetic field for orientation We performed indoor magnetic compass trials during the 2012 and 2013 fall migration seasons, in which individual monarchs collected from at least three different locations (see Methods) were tested in a flight simulator that was surrounded by a magnetic coil system used to vary the three different magnetic field parameters (horizontal, vertical, and intensity) ( Fig. 1a ). To facilitate flight in trials, they were conducted under diffuse white light conditions (spectrum: peak at 600 nm, range: 350–800 nm; total irradiance: 7.45 × 10 15 photons s −1 cm −2 ; Fig. 1b ), which also provided migrants with wavelengths of light that are crucial for a functioning magnetic sense in other insects [12] , [13] . 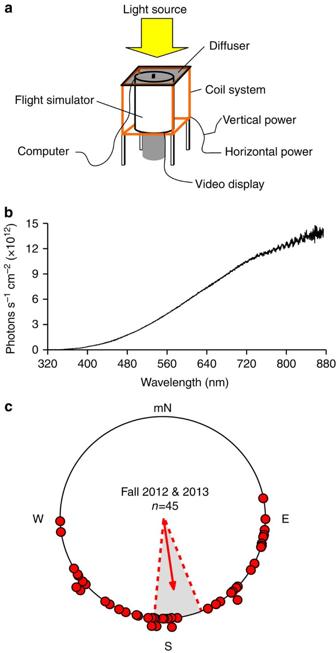Figure 1: Fall migrant monarch butterflies can use a magnetic field to orient in the proper southerly fall migratory direction. (a) Flight simulator and coil system used in magnetic compass trials. (b) Irradiance curve of lighting conditions during flight simulator trials. Light measurement was taken inside the flight simulator, with the flight encoder and diffuser in position, at the position of the head of the tethered monarch butterfly during trials. (c) Orientation of individual directional fall monarchs during the fall 2012 (n=18) and 2013 (n=27) migration seasons (red dots; both years pooled:n=45) in a generated field with a 45° inclination angle, at a 141 μT field intensity. For the circle diagram, arrow indicates mean group orientation, shaded area is 95% confidence interval, mN is magnetic north. Figure 1: Fall migrant monarch butterflies can use a magnetic field to orient in the proper southerly fall migratory direction. ( a ) Flight simulator and coil system used in magnetic compass trials. ( b ) Irradiance curve of lighting conditions during flight simulator trials. Light measurement was taken inside the flight simulator, with the flight encoder and diffuser in position, at the position of the head of the tethered monarch butterfly during trials. ( c ) Orientation of individual directional fall monarchs during the fall 2012 ( n =18) and 2013 ( n =27) migration seasons (red dots; both years pooled: n =45) in a generated field with a 45° inclination angle, at a 141 μT field intensity. For the circle diagram, arrow indicates mean group orientation, shaded area is 95% confidence interval, mN is magnetic north. Full size image Migrants from the 2012 and 2013 migratory seasons that were flown under artificial magnetic field conditions (inclination angle=45°; total magnetic field strength=141 μT) and that flew continuously for 5 min were significantly directional with a mean equatorward orientation (2012: α=162°, r =0.707, P =0.0001, n =18; 2013: α=179°, r =0.668, P =0.0001, n =27). There was no difference in orientation direction between years (Watson’s U 2 18, 27 =0.028, P >0.5), and the pooled orientation bearing was 172° ( r =0.676, P =0.0001, n =45) ( Fig. 1c ). The 5-min flight duration was previously found to be the minimal time required to evaluate directional orientation behaviour in individual butterflies in the flight simulator [6] . For assessing directionality in individual monarchs, we used a Z -value of ⩾ 500, as in previous publications [9] , [10] , [14] , [15] (see Methods). Z , which is the critical value of the Rayleigh test, is calculated by the equation: Z=nr 2 , in which n is the number of observations and r is the magnitude of the mean vector. Previous studies have shown, using reconstructed flight paths, that directional flight was apparent at Z ⩾ 500 and ambiguous at Z <500 (ref. 14 ); this Z -value parameter helped define the non-directionality of non-migrant, summer butterflies tested in the flight simulator outdoors under sunny skies. [14] Using the Z -value as a measure of directionality, we found that 87% of the 45 monarchs that flew continuously for 5 min exhibited a Z -value of >500. Accordingly, these 39 migrants provide a valid representation of the population of butterflies that flew. They were thus re-flown following the various trial perturbations outlined below with their first flight orientation values used as a control for comparison with subsequent experimental flight studies. Migrants have an inclination magnetic compass Most long-distance migratory animals studied to date use the inclination angle component of the Earth’s magnetic field to guide their latitudinal movement in either a poleward or equatorward direction [16] , [17] , [18] . We examined whether or not monarchs also have an inclination magnetic compass by testing the orientation behaviour of individuals when the vertical component of the field was inverted (−45°). This field manipulation alters the directional information provided by the inclination angle such that individuals would perceive it as a 180° shift [16] , [19] and is the acid test for the existence of an inclination compass [16] , [19] , [20] . Eight migrants (initial Z -values: 1,151.0±134.3, mean±s.e.m. ; Fig. 2a , left) re-flew for 5 min a second time under the same magnetic field conditions but with the inverted vertical component. The eight migrants re-flown continued to exhibit Z -values >500 (980.7±150.1) but displayed a grouped orientation towards magnetic North (α=1°, r =0.817, P =0.002, n =8; Fig. 2a , right) that was opposite (Moore’s test: R′ =1.418, P <0.001) from their initial group orientation ( α =175°, r =0.857, P =0.0008, n =8; Fig. 2a , left) by ~\n180°. These results demonstrate that individual fall migrants use the inclination angle of a magnetic field as a directional cue, suggesting that monarchs, like birds and sea turtles [16] , [17] , [18] , rely on an inclination compass for long-distance navigation. 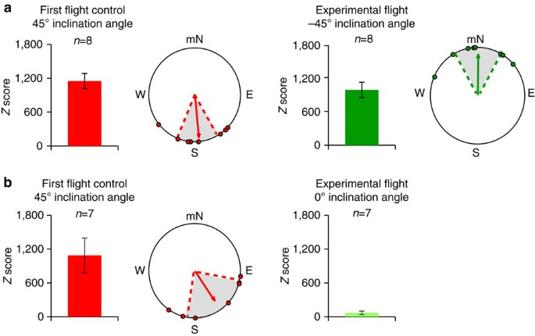Figure 2: The inclination magnetic compass of fall migratory monarch butterflies. (a) Fall migrant monarchs that oriented equatorwards during their initial flight (left; red;n=8), shifted their orientation towards magnetic North when tested a second time under similar generated field conditions (right; dark green;n=8), but with the inclination angle reversed (−45°). (b) Fall migrant monarchs that oriented equatorwards during their initial flight (left; red;n=7), each displayed flight with significantly reduced directionality (that is,Zscore <500) when tested a second time under a horizontal field (0° inclination angle) with the same field intensity (n=7). For bothaandb, bar graphs indicate the meanZ±s.e.m. score of animals for each group. Circular diagrams are the group orientation behaviour for each group in which each monarch plotted (dot) had aZscore >500. For each circular diagram, the arrow indicates mean group orientation, shaded area is 95% confidence interval, and mN is magnetic north. Figure 2: The inclination magnetic compass of fall migratory monarch butterflies. ( a ) Fall migrant monarchs that oriented equatorwards during their initial flight (left; red; n =8), shifted their orientation towards magnetic North when tested a second time under similar generated field conditions (right; dark green; n =8), but with the inclination angle reversed (−45°). ( b ) Fall migrant monarchs that oriented equatorwards during their initial flight (left; red; n =7), each displayed flight with significantly reduced directionality (that is, Z score <500) when tested a second time under a horizontal field (0° inclination angle) with the same field intensity ( n =7). For both a and b , bar graphs indicate the mean Z ±s.e.m. score of animals for each group. Circular diagrams are the group orientation behaviour for each group in which each monarch plotted (dot) had a Z score >500. For each circular diagram, the arrow indicates mean group orientation, shaded area is 95% confidence interval, and mN is magnetic north. Full size image Some animals use a polar compass for directionality and do not reverse their direction when the vertical component is inverted [21] , [22] . To rule out a potential contribution of a polar compass to directionality in migratory monarchs, we re-flew migrants at vertical field parameters mimicking those at the equator in which the inclination is 0° but still at a field strength of 141 μT; if the monarch’s magnetic compass is strictly inclinational, then directionality should be severely compromised with only the horizontal (polar) component present (that is, without a vertical component). The seven migrants that re-flew for 5 min under these conditions (initial Z -values 1,087.4±308.4 and group orientation of 146°, r =0.717, P =0.021, Fig. 2b , left) now exhibited a low degree of directionality, flying in circles, with Z scores <500 (69.1±30.9) ( Fig. 2b , right). Thus, the inclination magnetic compass is the dominant magnetic compass in monarchs, and the low Z scores represent the default state of orientation behaviour without the use of any inclination information. The inclination compass uses ultraviolet-A/blue light We next examined both the light sensitivity and spectral requirement of the inclination response. In migratory birds, the inclination compass is light-sensitive and thought to depend on radical pair-based chemical processes mediated by the flavoprotein cryptochrome (CRY) [16] , [18] , [23] . Given the ability of the two types of monarch butterfly CRYs to restore a light-dependent magnetic response in CRY-deficient Drosophila [12] , [13] , it is likely that monarchs also possess a light-dependent inclination compass. This was examined by using long-wavelength pass filters that transmitted wavelengths of light at >420 nm or >380 nm ( Fig. 3a ). Light intensity through the >420 nm filter was 6.76 × 10 15 photons s −1 cm −2 (91% of full-spectrum irradiance), while light intensity through the >380 nm filter was 6.82 × 10 15 photons s −1 cm −2 (92% of full-spectrum irradiance). These filters were used because the previous light dependence of the monarch CRY proteins for rescuing magnetosensitivity in CRY-deficient Drosophila was between 380 and 420 nm (ref. 13 ). When monarchs were exposed to light using the >420 nm filter, the five monarchs that flew for 5 min (initial Z values 985.2±150.1 and group orientation of 162°, r =0.866, P =0.014, Fig. 3b , left) each exhibited a low degree of directionality, flying in circles, with Z –values <500 (9.0±2.6) ( Fig. 3b , right); those orientation values were no different from those from migrants without a vertical component ( t 6 =1.6023, P =0.1602). When the >380 nm pass filter was used, allowing the addition of light between 380 nm and 420 nm, the five monarchs that flew for 5 min (initial Z -values 1,252.6±406.5 and group orientation of 202°, r =0.92, P =0.006, Fig. 3c , left) exhibited clear directionality with Z -values>500 (658.1±47.8 and group orientation of 157°, r =0.946, P =0.004, Fig. 3c , right). Thus, the monarch inclination compass appears to be light dependent with light in the ultraviolet-A/blue light spectral range (380 nm and 420 nm) important for inclination compass function. The >420 nm and >380 nm filters transmitted light intensities that were 91 and 92% of full-spectrum irradiance, respectively, yet each filter gave strikingly different orientation values. Hence, the contribution of decreased irradiance of the filters to the biological responses was negligible. The importance of light in the spectral range of 380–420 nm for compass function in monarchs is consistent with the inclination response being CRY dependent [13] . 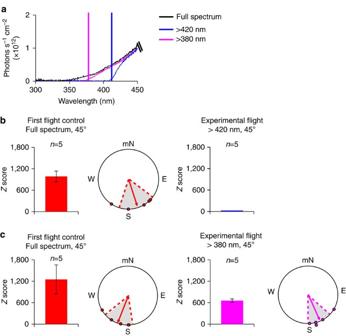Figure 3: The inclination magnetic compass uses ultraviolet-A/blue light. (a) Irradiance curves of lighting conditions during flight simulator trials. Black line indicates full spectrum light, blue line denotes filtered light that provided wavelengths of light >420 nm only, and purple line designates filtered light where only wavelengths of light >380 nm were available. (b) Migrants that oriented equatorwards during their first flight when tested under full spectrum lighting conditions (left; red;n=5) had significantly less directional flight, that is,Z<500 (right; blue;n=5), when tested under light that contained wavelengths >420 nm. (c) In contrast, monarchs that oriented equatorwards under full spectrum light during their initial flight (left; red;n=5), maintained similar oriented flight that was equatorwards when tested under lighting conditions that included wavelengths >380 nm (right; purple;n=5). For all trials, the inclination angle was 45° and the field intensity was 141 μT. In bothbandc, bar graphs indicate the meanZ±s.e.m. score of animals for each group. Circular diagrams consist of the group orientation behaviour for each group in which each monarch plotted (dot) had aZscore >500. In each circular diagram, arrow indicates mean group orientation, shaded area is 95% confidence interval, and mN is magnetic north. Figure 3: The inclination magnetic compass uses ultraviolet-A/blue light. ( a ) Irradiance curves of lighting conditions during flight simulator trials. Black line indicates full spectrum light, blue line denotes filtered light that provided wavelengths of light >420 nm only, and purple line designates filtered light where only wavelengths of light >380 nm were available. ( b ) Migrants that oriented equatorwards during their first flight when tested under full spectrum lighting conditions (left; red; n =5) had significantly less directional flight, that is, Z <500 (right; blue; n =5), when tested under light that contained wavelengths >420 nm. ( c ) In contrast, monarchs that oriented equatorwards under full spectrum light during their initial flight (left; red; n =5), maintained similar oriented flight that was equatorwards when tested under lighting conditions that included wavelengths >380 nm (right; purple; n =5). For all trials, the inclination angle was 45° and the field intensity was 141 μT. In both b and c , bar graphs indicate the mean Z ±s.e.m. score of animals for each group. Circular diagrams consist of the group orientation behaviour for each group in which each monarch plotted (dot) had a Z score >500. In each circular diagram, arrow indicates mean group orientation, shaded area is 95% confidence interval, and mN is magnetic north. Full size image The antennae likely contain relevant magnetosensors We next addressed the location of the magnetosensor. Previous work has demonstrated that the antennae of migratory monarchs are multimodal sensory organs that play an integral role for proper light-dependent, directional flight [3] , [9] , [10] , [15] . Accordingly, it is possible that the antennae also house the magnetoreceptors necessary for migratory monarchs to utilize the inclination angle of the Earth’s magnetic field. We thus re-tested first fliers under the inverted inclination angle conditions (−45°), but in which re-flown monarchs either had black-painted or clear-painted antennae for the second flight trial. The test condition was evaluated under the inverted inclination angle to rigorously examine the antennae as the potential source of the magnetosensor. Monarchs with black-painted antennae exhibited a low degree of directionality and flew largely in circles during this second flight ( Z =127.6±47.6; n =5) ( Fig. 4a , right) compared with the directionality of their first flights ( Z =1,231.3±181.2 and group orientation of 146°, r =0.826, P =0.024; Fig. 4a , left). The orientation values from migrants with black-painted antennae were no different from those from migrants without a vertical component ( t 10 =1.0818, P =0.3047). In contrast, monarchs with clear-painted antennae maintained Z -values >500 (clear-painted: 1,543.8±86.6, n =5 versus unpainted: 1,022.0±193.6, n =5) and were significantly oriented as a group towards magnetic North (α=345°, r =0.9, P =0.009, n =5; Fig. 4b , right) in a direction close to opposite (Moore’s test: R′ =1.332, P <0.001) from their initial group orientation in the direction of magnetic South ( α =209°, r =0.92, P =0.006, n =5; Fig. 4b , left). Remarkably, these data are consistent with the hypothesis that fall monarchs use a light-dependent, antenna-based inclination magnetic compass for directionality. 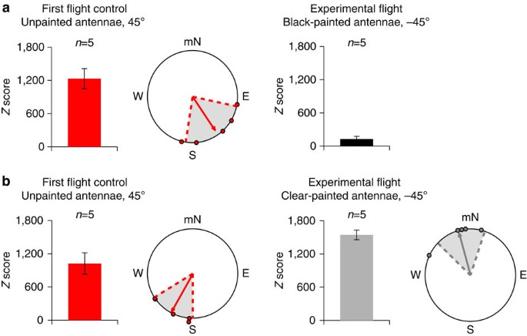Figure 4: The light-dependent magnetosensor involves the antennae. (a) Fall migrants that were oriented equatorwards during their initial flight (left; red;n=5) had significantly less directional flight (that is,Z<500) when both antennae were painted black during their second flight (right; black;n=5). (b) In contrast, fall migrants that were directed towards magnetic South during their initial flight (left; red;n=5) shifted towards magnetic North when tested with clear-painted antennae under reversed inclination angle conditions (right; grey;n=5). For bothaandb, monarchs (left diagrams; red) were tested in a generated field with a 45° inclination angle and an intensity of 141 μT. In contrast, monarchs (right diagrams; black foraand grey forb) were tested in a generated field that had the same intensity, but where the inclination angle was −45°. In bothaandb, each bar graph indicates the meanZ±s.e.m. score of animals for each group. Each circular diagram consists of the group orientation behaviour for each group in which each monarch plotted (dot) had aZscore >500. For each circular diagram, the arrow indicates mean group orientation, shaded area is 95% confidence interval, and mN is magnetic north. Figure 4: The light-dependent magnetosensor involves the antennae. ( a ) Fall migrants that were oriented equatorwards during their initial flight (left; red; n =5) had significantly less directional flight (that is, Z <500) when both antennae were painted black during their second flight (right; black; n =5). ( b ) In contrast, fall migrants that were directed towards magnetic South during their initial flight (left; red; n =5) shifted towards magnetic North when tested with clear-painted antennae under reversed inclination angle conditions (right; grey; n =5). For both a and b , monarchs (left diagrams; red) were tested in a generated field with a 45° inclination angle and an intensity of 141 μT. In contrast, monarchs (right diagrams; black for a and grey for b ) were tested in a generated field that had the same intensity, but where the inclination angle was −45°. In both a and b , each bar graph indicates the mean Z ±s.e.m. score of animals for each group. Each circular diagram consists of the group orientation behaviour for each group in which each monarch plotted (dot) had a Z score >500. For each circular diagram, the arrow indicates mean group orientation, shaded area is 95% confidence interval, and mN is magnetic north. Full size image The black paint itself was not the cause of the low degree of directionality ( Z -values <500) because previous outdoor studies of the time-compensated sun compass have shown that monarchs with black-painted antennae are each highly oriented ( Z -values >500), indicating that the sun compass has integrated skylight information (sensed though the eyes) for directionality [9] . However, because of the desychronized antennal clocks, the result of painting the antennae black, those migrants can no longer orient as a group in the proper flight direction. Intriguingly, without light input to the antennae and directional light cues for retinal processing, the migrants in the present study fly in circles, unable to find any directional cues, as light cues for both the sun compass and inclination compass are absent. In fact, this explains the low degree of directionality and circular orientation patterns that have been observed in another monarch flight simulator study in which individuals were exposed to the >420 nm long-wavelength filter outdoors with only blue sky visible [24] . The monarch inclination compass at Earth-strength fields Although exposure to a strong magnetic field can disorient migrant monarchs thereby suggesting that monarchs may possess a magnetic sense [25] , [26] , and even though animals that use a magnetic field for orientation can orient using a field that is considerably stronger than the Earth’s geomagnetic field [27] , we re-tested first fliers at a field intensity that fell within the range of the Earth’s geomagnetic field (25–65 μT) to determine if the inclination compass of migrants also functions at an Earth-strength field intensity. All re-flown migrants had Z scores >500 ( Fig. 5a , right; Fig. 5b ). We found that migrants that were oriented equatorward in trials at our stronger field intensity of 141 μT ( α =185°, r =0.681, P =0.033, n =7; Fig. 5a , left) were also similarly oriented equatorward (Moore’s test: R′ =0.474, P >0.5) when tested in a second flight trial occurring in a magnetic field with a 60° inclination angle, at an Earth-strength field intensity of 57 μT (α=173°, r =0.869, P =0.002, n =7; Fig. 5a , right). Furthermore, consistent with our results that tested migrants under reversed inclination angle conditions at 141 μT ( Figs 2a and 4b ), migrants that then flew for a third time in trials when tested at 57 μT but with a reversed inclination angle (−60°) switched their orientation behaviour towards magnetic North in a direction near opposite of their second (control) flight ( α =331°, r =0.892, P =0.01, n =5; Fig. 5b , right), in which the inclination angle was 60°. Moreover, the orientations of the second control flight (57 μT; 60° inclination angle) and third flight of migrants (57 μT; −60° inclination angle) were significantly different from each other (Moore’s test: R′ =1.279, P <0.005). Taken together, these data demonstrate the ability of migrant monarchs to use an inclination compass to orient in the proper equatorward migratory direction, which includes conditions at an Earth-strength field intensity and at an inclination angle encountered during their journey south. The data support the idea that monarchs can use an inclination compass during their actual fall migration in the wild. 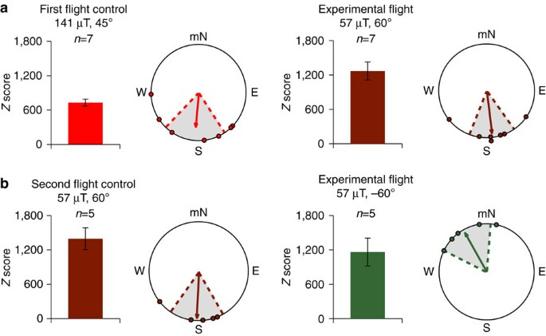Figure 5: The inclination compass of monarchs functions at an Earth-strength field intensity. (a) Orientation of individual directional monarchs (left; red;n=7) in a generated field with a 45° inclination angle, at a 141 μT field intensity. The orientation of individual directional monarchs (right; maroon;n=7) tested a second time (same monarchs from left circular diagram), but in a generated field with a 60° inclination angle, at a 57 μT field intensity. (b) Monarchs that flew towards magnetic South (left; maroon;n=5) in a field with a 60° inclination angle and a 57 μT intensity (second flight) reversed their flight orientation to magnetic North (right; green;n=5) in a generated field with a −60° inclination angle at a 57 μT field intensity, when tested a third time (same monarchs from left circular diagram). In bothaandb, circular diagrams consist of the group orientation behaviour for each group in which each monarch plotted (dot) had aZscore >500. In each circular diagram, the arrow indicates mean group orientation, shaded area is 95% confidence interval, and mN is magnetic north. For bothaandb, bar graphs indicate the meanZ±s.e.m. score of animals for each group. Figure 5: The inclination compass of monarchs functions at an Earth-strength field intensity. ( a ) Orientation of individual directional monarchs (left; red; n =7) in a generated field with a 45° inclination angle, at a 141 μT field intensity. The orientation of individual directional monarchs (right; maroon; n =7) tested a second time (same monarchs from left circular diagram), but in a generated field with a 60° inclination angle, at a 57 μT field intensity. ( b ) Monarchs that flew towards magnetic South (left; maroon; n =5) in a field with a 60° inclination angle and a 57 μT intensity (second flight) reversed their flight orientation to magnetic North (right; green; n =5) in a generated field with a −60° inclination angle at a 57 μT field intensity, when tested a third time (same monarchs from left circular diagram). In both a and b , circular diagrams consist of the group orientation behaviour for each group in which each monarch plotted (dot) had a Z score >500. In each circular diagram, the arrow indicates mean group orientation, shaded area is 95% confidence interval, and mN is magnetic north. For both a and b , bar graphs indicate the mean Z ±s.e.m. score of animals for each group. Full size image As fall migratory monarchs have been observed to maintain a constant southwards flight direction under dense cloud cover conditions [11] , it has been hypothesized that fall migrants may use geomagnetic cues for directionality, when directional daylight cues are unavailable to them during migration [3] , [11] . Previous studies examining the existence of a magnetic compass in migratory monarchs, however, have yielded weak, conflicting results. For example, although work has shown that monarchs can become disoriented when exposed to experimentally generated strong magnetic fields [25] , [26] , other work using a flight simulator found that migrants do not fly in an oriented manner when tested using simulated overcast skies, under either artificial or ambient magnetic fields [5] , [28] . The defined spectral requirement for the inclination compass discovered in our studies potentially explains why previous flight simulator studies were unable to identify an inclination magnetic compass. In one of those studies [28] , it is clearly stated that the test lighting conditions (consisting of a milky-white, non-UV-transmitting, translucent Plexiglas lid) excluded UV-A/blue light. Because both flight simulator studies were from the same group, it is likely that the lighting conditions of the other study [5] also excluded the relevant spectral feature for detecting the use of an inclination compass. Moreover, given that we observed the use of an inclination magnetic compass by individuals that were tested in different years, sampled from at least three different locations, and tested at different magnetic field intensities, strengthens the idea that the spectral requirement is what is necessary for a functioning magnetic sense in monarch butterflies. To our knowledge, our work is the first demonstration of the use of an inclination magnetic compass by a long-distance migratory insect. Our data suggest that the inclination compass may facilitate the fall migratory journey to the overwintering sites (that is, migrants respond to the sign of the inclination angle and respond by flying equatorward with a positive inclination angle as seen in our results), in a similar and/or concurrent manner as the time-compensated sun compass, or serve as a calibrator or backup mechanism to the sun compass [3] . Whether or not migrants possess a geomagnetic map sense that allows them to recognize or locate specific locations (for example, overwintering sites) as observed in sea turtles [29] , [30] remains to be determined, however. The data also suggest that the antennae may contain the light-sensitive magnetosensors for the light-dependent inclination compass, thereby providing an additional migration-relevant function for the antennae of monarch butterflies. Involvement of the eyes and/or the brain in magnetosensing in migrant butterflies has not been ruled out. Knowledge of the presumed location of the relevant light-sensitive component of the magnetosensor in monarchs opens the way for evaluation of both the molecular and genetic mechanisms of magnetoreception [31] , [32] and the involvement of their CRYs [12] , [13] . Taken as a whole, our study reveals another fascinating aspect of monarch butterfly migratory behaviour. Greater knowledge of the mechanisms underlying the fall migration may well aid in its preservation, currently threatened by climate change and by the continuing loss of milkweed and overwintering habitats. Another vulnerability to now consider is the potential disruption of the magnetic compass in monarchs by human-induced electromagnetic noise, which can apparently disrupt geomagnetic orientation in a migratory bird [33] . Animal rearing and housing In 2012, fall migratory monarch butterflies were captured by Fred Gagnon (between 1 September 2012 and 22 September 2012) near Greenfield, Massachusetts (latitude 42°59′N, longitude 72°60′W). In 2013, fall migratory butterflies were captured by Fred Gagnon (between 1 September 2013 and 28 September 2013; near Greenfield, Massachusetts), Carol Cullar (10 October 2013; near Eagle Pass, Texas [latitude 28°51′N, longitude 100°53′W]), and David Cook (30 October 2013; near St. Marks, Florida [latitude 30°9′N, longitude 84°12′W]). After capture, migrants were housed indoors in glassine envelopes in a Percival incubator under fall-like conditions: a light:dark cycle (LD) set to prevailing light conditions (12 h:12 h LD, 0600–1800 Eastern Standard Time), a constant temperature of 21 °C during the light phase and a constant 12 °C during the dark period, and 70% humidity. Flight simulator trials and analysis Monarchs were housed under fall-like conditions for at least 10 days before testing. Monarchs of mixed sex were tethered for flight trials as previously described, and their flight behaviour was assayed with a flight simulator [9] , [10] , [15] . Flight direction was recorded by computer configured to record the direction of flight every 200 ms. Flight simulator trials for both fall 2012 and 2013 were conducted indoors at the University of Massachusetts Medical School (Worcester, Massachusetts: latitude 42°28′N, longitude 71°76′W), between 1100 and 1630 EST. Migrants were held in a non-metallic holding cage positioned within the coil system (see below) for 1 h before testing in the flight simulator, to acclimate them to the generated magnetic field [27] and to trial conditions [9] , [10] , [15] . To facilitate flight during trials, the flight simulator was illuminated from above ( Fig. 1a ) by diffuse white light (Utilitech 250W no. 0320778; spectrum: peak at 600 nm, range: 350–800 nm; intensity: 7.45 × 10 15 photons s −1 cm −2 ; Fig. 1b ), which also provided migrants with wavelengths of light that are critical for a functioning magnetic sense in other insects [12] , [13] . A diffuser was positioned in the light path, directly on top of the opening of the flight simulator [7] ( Fig. 1a ). Irradiance measurements (using an Ocean Optics USB 2000 fiber optic spectrophotometer) were taken inside the flight simulator, with the flight encoder and diffuser in position, at the position of the head of the tethered monarch butterfly during trials. The flight simulator was surrounded by a Helmholz coil system ( Fig. 1a ) that was used to control the magnetic field in which an individual butterfly was tested. The coil system consisted of two independent two-coil systems arranged orthogonally, with each coil powered by its own power supply, and constructed in accordance with coil system designs used previously [34] . One coil was used to control the horizontal component of the magnetic field, and this coil was aligned with the north-south magnetic axis. The second coil was used to control the magnetic field’s vertical component [34] . Magnetic field parameters at the position of the tethered monarch during flight simulator trials (horizontal and vertical field components) were measured using an Applied Physics Systems tri-axial fluxgate magnetometer (model 520A). Using these values, the inclination angle and total field intensity were calculated for each magnetic field condition. The flight behaviour of monarchs was monitored on a video screen during trials, as well as recorded onto DVD. The behaviour of monarchs during trials was recorded for 82 out of 92 trials (for the 10 unrecorded trials, the DVD recorder malfunctioned, for example, the DVD became full during a trial that prevented the trial from being recorded). Two independent observers, unaware of the flight treatment (for example, first flight control or experimental condition), the magnetic field used during trials, and the antennal condition of migrants (for example, black- or clear-painted antennae), monitored recorded trials and verified the flights of butterflies (for example, flight >5 min) in the flight simulator. For all conditions, we determined the significance of flight orientation and the mean direction of monarchs tested in the flight simulator using circular statistics (for example, Rayleigh’s test for both individual and mean group orientation, Watson U 2 test for unpaired group comparisons, Moore’s test for paired group comparisons) in Oriana (Kovach Computing Services). Z score analysis Because Z score is sample size dependent, butterflies from each group and under each condition (18 control and treatment groups) that were used in all of the comparisons in our study (12 statistical comparisons) were flown for the same amount of time and therefore any observed differences in Z scores were not simply the result of differences in flight times. There were no differences in the mean flight time values between groups in each of the comparisons that we made in our analyses (all P -values for each comparison were non-significant, the Bonferroni corrected α =0.0042 for 12 statistical tests). The following are the flight times in seconds (mean±s.e.m., number of animals in each group) for each group used in our comparisons: Fall 2012 first flights: 429.7±23.9, 18; Fall 2013 first flights: 407.8±20.9, 27; inclination angle control group: 464.9±41.5, 8; inclination angle test group: 346.9±24.7, 8; horizontal field control group: 347.1±19.1, 7; horizontal field test group: 324.7±9.0, 7; 420 nm control group: 392.6±56.8,5; 420 nm treatment group: 318.24±0.31, 5; 380 nm control group: 373.64±57.3, 5; 380 nm treatment group: 351.44±20.7, 5; black-painted control group: 507.84±57.98, 5; black-painted treatment group: 343.64±13.2, 5; clear-painted control group: 426.2±52.52, 5; clear-painted treatment group: 458.88±58.31, 5; Earth-strength control group: 396.47±24.48,7; Earth-strength treatment group: 505.37±36.39, 7; Earth-strength inclination control group: 519.96±29.60, 5; Earth-strength inclination treatment group: 383.64±23.42, 5. Testing for magnetic sensitivity in monarchs To first assay for a magnetic response in migrants, after a 1-h acclimation period to the generated magnetic field (inclination=45°; total magnetic field strength=141 μT), we observed the flight behaviour of individual butterflies in flight simulator trials during fall 2012 and 2013. Only monarchs that flew continuously (>5 min) [9] , [10] , [15] were considered for analysis, and we found no difference in the flight behaviour of monarchs between years (Watson’s U 2 18, 27 =0.028, P >0.5). Out of the 171 monarchs tested during fall 2012 and 2013, 45 flew >5 min during their first flight. This 26% success rate of migrants tested indoors in our trials is similar to the success rate of monarchs that flew continuously for 5 min during their first attempt in outdoor flight simulator trials (31% success rate; 34 out of 110 monarchs in fall 2010 (ref. 15 )) (Fisher’s exact test, P =0.4174), as well as outdoor flight release trials that yielded useable flight data (35% success rate; 23 out of 66 monarchs [15] ) (Fisher’s exact test, P =0.2031). Of these 45 fliers, 39 flew directionally ( Z score >500): this 87% rate of individual directionality was similar to the rate of individual directional fliers previously observed in outdoor flight simulator trials (92%, 46 out 50 migrants [10] ) (Fisher’s exact test, P =0.5095). These monarchs that demonstrated significant directional flight behaviour ( Z score >500) during their first flight were then used in our subsequent experiments (see below). Within each experimental group, each monarch was only tested once. To minimize the use of monarchs, some butterflies were tested in more than one treatment group. For each treatment, monarchs were acclimated to trial field conditions for 1 h before testing, and only monarchs that flew >5 min were used in analysis. Testing for the use of an inclination compass To test for the use of an inclination compass, monarchs were then tested a second time under similar generated magnetic field conditions as during their first flight, but where we reversed the inclination angle (−45°) by reversing the vertical component of the field, using our vertical coil system (horizontal component remained unchanged). All re-fliers during this second trial ( n =8) that flew for the required 5 min were directional ( Z score >500). To confirm the use of an inclination compass and to rule out the potential use of polarity for directionality, we tested another set of monarchs a second time under field conditions in which the inclination was 0° but still at a field intensity of 141 μT (that is, a horizontal field with the same total field intensity as that of the first flight control). All re-fliers that flew for the required 5 min ( n =7) under this horizontal field exhibited significantly reduced directionality ( Z score <500) in comparison with their first flight. Testing spectral requirement of the inclination compass To determine whether a working inclination compass requires the presence of specific wavelengths of light, we re-tested monarchs after their first flight under filtered light conditions. Monarchs were re-tested under first flight magnetic field conditions (inclination angle=45°; total field intensity=141 μT), but where light consisted of wavelengths of either >420 nm or >380 nm (long-wavelength filters E420 and E380 from Gentex). For each of these filtered light conditions, we had five monarchs that flew >5 min. All five monarchs that flew under >420 nm lighting conditions had significantly reduced directionality ( Z scores <500) relative to the first control flight; in contrast, all five monarchs that flew under >380 nm lighting conditions had similar directionality ( Z scores >500) as their first control flight. Locating the putative magnetosensor in monarchs To determine whether the inclination compass of migrants consists of a light-dependent, antenna-based mechanism, migrants were re-tested after their first flight trial (inclination=45°; total magnetic field strength=141 μT), but where butterflies either had both antennae painted black ( n =5) or clear ( n =6) during this second trial (field conditions were as during their first flight but with a reversed inclination angle, −45°). Black paint was used to prevent the sensing of light by the antennae, while clear paint was used as a control for the painting process, as clear paint still permits the antennae to receive light [9] , [10] , [15] . Antennal painting has no effect on flight motivation or capability in monarchs [9] , [10] , [15] . During this second flight, 10/11 monarchs flew >5 min (5 black-painted, 5 clear-painted). Here, all monarchs with black-painted antennae had significantly reduced flight directionality relative to the first control flight ( Z score <500), whereas all monarchs with clear-painted antennae had similar flight directionality as their first flight ( Z score >500). Inclination compass at Earth-strength magnetic conditions To determine whether the inclination compass of migrants functions at Earth-strength field intensities, we compared the first flights of monarchs under our stimulus of 141 μT (45° inclination angle), which is stronger than that of the Earth’s geomagnetic field (25–65 μT), with a second flight using a generated magnetic field with a field intensity (57 μT) that fell within that of the Earth’s. We initially aimed at presenting migrants with a magnetic field that had a field intensity and inclination angle that was consistent with the geographical location of trials, but, due to limitations with the testing room (that is, a slightly higher than ambient horizontal component), we were unable to do so. Regardless, using our coil system, we were able to produce a magnetic field with an intensity within the range of the Earth’s natural field, with an inclination angle (60°) that corresponded to an inclination angle that actual migrating monarchs will encounter during their journey to their overwintering sites (that is, 60°=Waco, Texas; National Oceanic and Atmospheric Administration National Geophysical Data Centre, http://www.ngdc.noaa.gov/ngdc.html ). We had 7 migrants that flew for >5 min under these Earth-strength field conditions (57 μT with a 60° inclination angle), and all of them flew directionally ( Z score >500). These seven migrants were then tested a third time, but where the inclination angle (−60°) of the Earth-strength field was reversed during trials using our coil system. Under these conditions, five out of seven migrants (71%) flew >5 min. All five of these fliers flew directionally ( Z score >500). How to cite this article: Guerra, P. A. et al . A magnetic compass aids monarch butterfly migration. Nat. Commun. 5:4164 doi: 10.1038/ncomms5164 (2014).